Direct stereoselective α-arylation of unmodified enals using an organocatalytic cross-coupling-like reaction Cross-coupling reactions typically rely on the use of transition metal catalysis. However, although achieving this process using metal-free organocatalysts is highly challenging, it could offer unique opportunities to discover novel bond-forming strategies in organic synthesis. Here we report a new amine catalysed direct stereoselective C-H α-arylation reaction of unmodified enals with bromoarenes. The power of this process, which involves an unprecedented iminium-Michael-alkylation-enamine-retro-Michael cascade sequence, has been demonstrated in the context of direct α-functionalization reactions of simple, unmodified enals with 4-bromophenols, 1-bromo-2-naphthol and 3-bromoindoles under mild reaction conditions. Notably, the process can be used for highly stereoselective syntheses of non-readily accessible E isomers, which normally require the use of transition metal-promoted cross-couplings and functionalized enals. The results of these studies significantly expand the scope of aminocatalysis. Cross-coupling reactions have revolutionized chemical synthesis and, arguably, have become one of the most powerful tools for carbon–carbon bond formation [1] , [2] , [3] , [4] , [5] , [6] . In recent years, the scope of cross-couplings have moved beyond traditional processes by enabling direct arylation reactions of aromatic C–H bonds [7] , [8] , [9] , [10] , [11] , [12] , [13] , [14] , [15] . Although great strides have been made in the development of efficient methods for coupling and direct arylation reactions, the strategies devised to date rely on transition-metal-assisted approaches for which new transition metal complexes and ligands have been developed. Moreover, owing to the general unreactivity of C–H bonds, harsh reaction conditions (for example, strong base used and at high temperature) are generally required to promote transition-metal-catalysed direct crossing couplings and difficulties associated with the control of chemo-, regio- and stereoselectivity are often problematic. The pioneering work on respective enamine and iminium catalysis by List and Barbas [16] , [17] and MacMillan [18] , [19] , [20] serve as the conceptual basis for the field of organocatalysis. A large number of unprecedented and typically stereoselective organic transformations, which are complementary to transition-metal catalysed processes, have been devised using this chemistry. The success of aminocatalysis can perhaps be attributed to the involvement of unique activation modes that enable stereoselective reactions to proceed under mild conditions and with a broad functional compatibility and operational simplicity. Although the main focus in this area will continue to be the design of highly efficient catalysts that promote existing reactions with greater turnover numbers [21] , [22] , expansion of the scope of aminocatalysis to include new reactions is an important yet challenging aim. To our knowledge, the exploration of organocatalysis in the arena of cross-coupling reactions has not been described previously. Interest in functionalized α,β-unsaturated aldehydes has grown significantly in recent years because of the results of their broad utility in cosmetic [23] , [24] , pharmaceutical [25] , [26] , [27] , [28] , [29] , [30] and agrochemical [31] , [32] , [33] , [34] industries. Moreover, enals are arguably the most widely used substrates in current organocatalytic reactions [18] , [19] , [20] . Therefore, efficient methods for the generation of structurally diverse α,β-unsaturated aldehydes with high levels of E / Z stereoselectivity (especially E -selective synthesis of α-substituted enals) are highly desirable ( Fig. 1 ). Although cross-aldol condensation reactions of two different aldehydes afford facile access to these targets, intrinsic problems associated with poor E / Z stereoselectivity, in which formation of thermodynamically more stable Z isomers are favoured, and production of complex product mixtures render this process impracticable [28] . State-of-the-art approaches to these targets use Pd(0)-catalysed cross-coupling protocols, including Suzuki–Miyaura reaction of potassium aryl trifluoroborates with alkenyl bromides ( Fig. 1a ) [35] and the reaction of benzyl bromides with diazoesters ( Fig. 1b ) [36] . 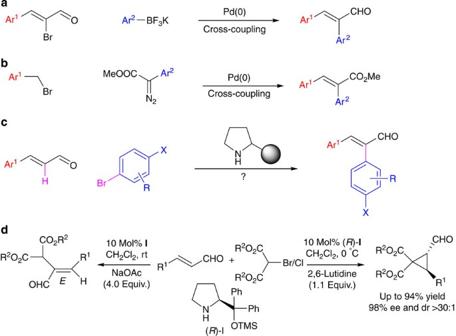Figure 1: Approaches to selective (E)-α-arylation of enals and acrylates. (a,b) Pd-catalysed cross-couplings for introducing aryl groups at α-postion at enals and acrylates. (c) Organocatalytic direct α-arylation of unmodifed enals. (d) An organocatalytic Michael-alkylation cascade. Figure 1: Approaches to selective ( E )-α-arylation of enals and acrylates. ( a , b ) Pd-catalysed cross-couplings for introducing aryl groups at α-postion at enals and acrylates. ( c ) Organocatalytic direct α-arylation of unmodifed enals. ( d ) An organocatalytic Michael-alkylation cascade. Full size image In recent years, we have carried out investigations leading to the development of new organocatalysed reactions and, in particular, those that involve efficient and stereoselective cascade processes [37] . These atom-economical processes serve as powerful approaches to transform readily available chemicals in one-pot operations to useful building blocks for organic synthesis. This effort has recently resulted in the discovery of an organocatalytic, enantioselective Michael-alkylation cascade sequence in which chiral propanes are generated from enals and bromomalonates ( Fig. 1d ) [38] , [39] . In this study, an unexpected side reaction was uncovered that produces stereoselectively ( E )-α-substituted malonate enals. The results from ensuing mechanistic studies revealed that this product is formed through a catalytic Michael-alkylation sequence that gives rise to a cyclopropane intermediate, which then undergoes a stereospecific ring-opening via an enamine-initiated retro-Michael reaction. Stimulated by these findings, we question whether this chemistry could serve as the foundation of a new transformation involving a Friedel–Crafts alkylation-ring opening cascade ( Fig. 1c ). If successful, this process would give products derived by direct connection of the α-carbon of an enal with an aryl-ring carbon. To our knowledge, no transformation of this type exists for direct 'coupling' of unmodified enals with arenes. Here we describe the observation made in an investigation leading to the development of an amine catalysed, direct, stereoselective α-arylation of unmodified α,β-unsaturated aldehydes with brominated aromatics that takes place through an unprecedented 'cross-coupling-like' process ( Fig. 1 ). The observations show that by using the methodology, a variety of brominated phenols and indoles an be efficiently converted under mild reactions conditions to ( E )-α-substituted enals. Substrate design A consideration of the proposed Friedel–Crafts alkylation-ring opening pathway led to the conclusion that the aromatic substrates that participate as Michael donors in the process must be electron rich so that the initial electrophilic aromatic substitution step can occur efficiently. Although organocatalytic Michael addition reactions of electron-rich aromatic compounds to α,β-unsaturated aldehydes has been intensively studied [40] , [41] , to our knowledge no precedent exists for bond formation at ipso -positions, which is an essential component of the new α-arylation reaction. In typical transition-metal-catalysed cross-coupling reactions, the halo-substituent not only polarizes the C–X bond for oxidative insertion of the transition metal, it also functions as a leaving group in the reductive elimination step. In the new 'cross-coupling like' process, the aromatic ipso -halogen functions in a similar manner in that it serves as a leaving group in the ensuing alkylation step. More importantly, it functions as an appropriate pool to balance both steric and electronic effects that govern the initial Michael addition process. On the basis of these considerations, we reasoned that bromine would serve optimally in both capacities in that its steric hindrance would be compensated by its electron-donating ability as well as its softness, which would favour conjugated addition. Accordingly, p -bromophenol was selected as the substrate in our exploratory investigations of the new process. Optimization of reaction conditions A model cross-coupling-like reaction at room temperature between p -bromophenol ( 1a ) and trans-p -nitro-cinnamaldehyde ( 2a ) in the presence of Na 2 CO 3 and the catalyst diphenylprolinol TMS ether I was explored in our initial effort ( Table 1 ) [38] , [39] . Indeed, the reaction occurs to give the desired product 3a , but in only a moderate yield. Ensuing studies showed that the efficiency of formation of this product was highly solvent dependent (entries 1–9). Importantly, reaction in chloroform occurs in yields as high as 41% in a highly stereoselective manner (>30:1 E/Z ratio; entry 9). In contrast, reactions taking place in other solvents, such as acetonitrile, dimethylformamide and dimethylsulfoxide, occur with low yields even when prolonged reaction times are used. A survey of the other amine catalysts II – VII do not lead to favourable results (entries 10–15). Moreover, elevating the temperature of the reaction in chloroform to 60 °C shortens the reaction time significantly without affecting the yield (entry 16). As expected, when Cl or I are used as leaving groups (entries 17 and 18), the reaction does not take place as efficiently as in Br. Probing base additives lead to the conclusion that Na 2 CO 3 is optimal (entries 19 and 20) and an increase in the amount of 2a from 2.0 to 4.0 equiv results in an improvement of the reaction yield (entry 21). These results suggest that addition of 2a via a syringe pump over a 7-h period would improve yields, a proposal that is supported by the observation that the efficiency of the process is enhanced (85% yield, entry 22) when slow addition of 2.0 equiv of 2a is used. Reducing the catalyst loading results in slower transformation due to slow catalyst turnover, and thus longer reaction time is needed, generally observed in covalent-bond-mediated aminocatalysis. However, in our cases, under the reaction conditions at relatively high temperature (65 °C), although longer reaction time could completely consume the starting materials, the reaction become more complicated with unidentified by-products formed and therefore even lower reaction yields are obtained. As seen, when 10 and 5 mol% catalyst loadings used, it takes respectively 2 days and 3 days for complete conversion. However, only 39 and 12% yields of desired product 3a are obtained, respectively ( Table 1 , entries 23 and 24). Table 1 Optimization of amine-catalysed direct α-arylation reaction of trans-p -nitro-cinnamaldehyde with p -halogenated phenols * . Full size table Scope of α-arylation reactions of enals The scope of the α-arylation reactions of p -bromophenols with enals is probed using the optimized conditions described above. 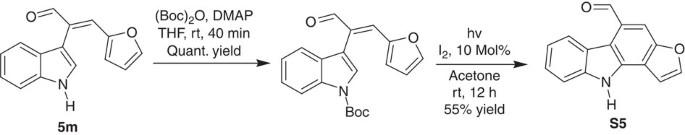Figure 2 Synthesis of furocarbazoleS5via photoelectronic cyclization-photoinduced decarboxylation cascade process. As the results in Table 2 show, the I -catalysed 'cross-coupling-like' reaction displays broad substrate compatibility. Reactions of a variety of structurally diverse cinnamaldehydes, in which the aromatic ring bears electron-withdrawing, electron-neutral and electron-donating substituents, with p -bromophenol 1a as a Michael donor, were explored (entries 1–17). These transformations take place smoothly to give products 3 in moderate to excellent yields (46–99%). The E configuration of the products is assigned based on a single X-ray crystallographic analysis of 3a (CCDC-844422, see Supplementary Fig. S1 and Supplementary Data 1 ). Table 2 Scope of amine-catalysed direct α-arylation reactions of p -boromophenols with enals * . Full size table The general conclusion drawn from the results of this effort is that steric effect on reactivity and stereoselectivity are more pronounced than that of electronic effects. For example, relatively lower yields and poorer E / Z ratios attend reactions of cinnamaldehydes containing ortho - and meta - versus para -aromatic substituents (entries 6–8 and 12–13 versus entries 1–5 and 9–11). The steric effect also reflects in the reaction of even more hindered β,β-disubstituted enals (for example, trans -3-phenyl-but-2-enal): no reaction takes place at all. Moreover, in general, reactions of electron-withdrawing-substituted cinnamaldehydes yield products in relatively higher yields and E/Z selectivities. In addition, the process can be extended to heterocyclic and conjugated arenes (entries 14–16). Finally, the results show that an aliphatic enal does not react to give the desired product (entry 17). Nevertheless, interestingly, an unexpected 4-methylbenzaldehyde is obtained in 64% yield. The product is presumably through a [3+3] process [42] . The effects of varying the substitution pattern (for example, at positions 2, 3 and 6) of the p -bromophenol reactants are also investigated ( Table 2 , entries 18–23). The results show that p -bromophenol substituents have only a limited influence on yields and stereoselectivities. In general, good to high yields (62–99%) and high E / Z selectivities are observed in all cases. As expected, electron-donating groups are found to facilitate the process (entries 18–20 versus 21–23), whereas the effect of sterics is limited. Finally, we also find that reactions of substrates, in which the phenol –OH group is changed to –OMe, NH 2 , NHMe, NMe 2 and SH, do not take place (data not shown). We also probe 2-bromophenol for the reaction. No reaction occurs and only starting materials are recovered. It is believed that 2-bromophenol is more crowded than 4-bromophenol for the cross-coupling process. Such an effect becomes significant in the initial Michael addition reaction, which is very sterically sensitive, as results of the generation of a highly crowded quaternary carbon centre and requires high energy for dearomatization. However, we find that if 1-bromo-2-naphthol, which is considered as an analogue of 2-bromophenol, is used as a Michael donor, we do observe the formation of the desired product. Under optimized reaction conditions (in MeCN, NaOAc, 60 °C, 3 days) in 'one-pot' operation, we obtain the desired coupling E -product in 56% yield and with an excellent E:Z ratio (>30:1). The driving force for the occurred process is presumably due to the higher reactivity of less aromatic 1-bromo-2-naphthnol. The success of the I -promoted direct α-arylation of enals with p -bromophenols prompts us to explore the ability of non-phenolic substrates to serve as aromatic coupling partners. We envision that 3-bromoindoles would be good substrates for the reaction as they are electron-rich species and they have been used in organocatalysed enantioselective Friedel–Crafts reactions [41] . Furthermore, functionalized indoles are important building blocks in organic synthesis and 'privileged' structures in drug discovery [43] . 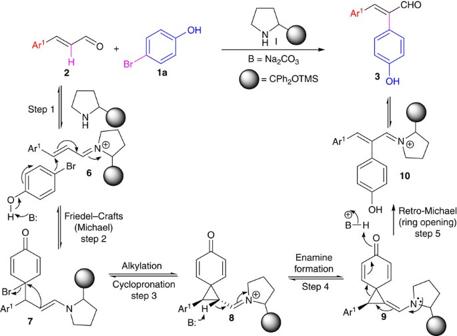Figure 3 A proposed reaction mechanism for α-arylation reactions of enals with 4-bromophenol. The results of extensive exploratory and optimization studies of the model reaction between 3-bromoindole ( 4a ) with trans-p -nitro-cinnamaldehyde ( 2a ) revealed that catalyst I , CHCl 3 as solvent at 60 °C, and NaOAc, instead of Na 2 CO 3 , represent optimal conditions ( Table 3 , entry 1 and Supplementary Tables S1 and S2 for details of optimization processes). It is noteworthy that, in contrast to reactions of 4-bromophenols, the process can be performed in one pot without the need for gradual addition of the 3-bromoindoles. Table 3 Scope of amine-catalysed direct α-arylation reactions of 3-bromoindoles with enals * . Full size table The scope of I -catalysed direct α-arylation reactions of 3-bromoindoles ( 4 ) with enals ( 2 ) is examined ( Table 3 ). The results show that the processes serve as a general and efficient method to prepare a variety of ( E )-α-indole-enals. The E configuration of products is assigned based on a single X-ray crystallographic analysis of 5a (CCDC-844421, see Supplementary Fig. S2 and Supplementary Data 2 ). Notably, high yields (65–100%) and good to high E -selectivities (9:1 to >30:1) attend these processes. Furthermore, the reactions generally proceed faster and with higher yields and E -stereoselectivities than those with 4-bromophenols. In addition, as observed with reactions of 4-bromophenols, electron-withdrawing (entries 1–6), electron-neutral (entry 7) and electron-donating substituents (entries 8–11) or a combination (entry 12) on enals ( 2 ) are found to have limited effects on these processes. Reactions of 3-bromoindoles also occur in high yields with other heterocycles (entry 13) and with other conjugated aromatic systems (entries 14–15). Again, steric effects are found to influence the efficiency of these reactions more than electronic effects. In general, more hindered substrates react with diminished E /Z selectivities (entries 4–6, 10–11 and 15). A survey of the structural tolerance of 3-bromoidoles indicates that, in all cases, good to high yields (65–100%) and high stereoselectivities (16:1 to >30:1) are achieved (entries 16–20), regardless of the size and electronic characteristics of substituents. Interestingly, in case of 5-methoxyindole (entry 20), a 2-brominated product is unexpectedly obtained. The ( E )-α-indolyl-β-arylacrylaldehydes 5 can serve as valuable precursors for the efficient synthesis of [α]-annulated carbazoles, an important class of compounds with fascinating biological properties such as anti-tumour, anti-microbial and anti-fungal activities [44] . Moreover, recently, their application has been expanded to the areas of molecular imaging and material chemistry [45] , [46] . As demonstrated, for instance, compound 3m can be efficiently transformed to furocarbazole S5 through a photoelectronic cyclization-photoinduced decarboxylation cascade ( Fig. 2 ). Furocarbazole S5 and its analogues are of considerable biological interest. They can be potentially used for the treatment of various infections and poisonous snake bites [47] . Figure 2 Synthesis of furocarbazole S5 via photoelectronic cyclization-photoinduced decarboxylation cascade process. Full size image Cross-coupling reactions are typically performed by using transition-metal catalysis. Only recently did Sun et al . [48] and Lei [49] independently describe elegant organocatalysed cross-coupling reactions of aryl iodides/bromides with arenes using 1,10-phenanthroline and N , N' -dimethylethane-1,2-diamine as respective catalysts in the presence of t -BuOK. It is believed that these processes take place through radical pathways [48] , [49] , [50] , [51] , [52] , [53] . The strategic basis of the new coupling reactions described above are completely different from those reported by Sun et al . [48] , Lei [49] and others [50] , [51] , [52] , [53] . The proposed mechanism of the amine I catalysed α-arylation reactions of enals ( Fig. 3 ) involves the intermediacy of iminium ion 6 , derived from the reaction of enal 2 with catalyst I followed by a Friedel–Crafts (or Michael addition) reaction with, for example, 4-bromophenol 1a . This step is key to success of the overall process, as it must not only take place smoothly to initiate subsequent steps but, more importantly, it must occur regioselectively at a highly crowded para -phenol position. Therefore, the facility of the electrophilic aromatic substitution step requires the presence of an appropriately small halogen, like Br, with a weaker C–X versus C–C bond and an electron-donating or weak-withdrawing capacity. Figure 3 A proposed reaction mechanism for α-arylation reactions of enals with 4-bromophenol. Full size image Importantly, as mentioned above, to the best of our knowledge, no precedent exists for an organocatalysed Friedel–Crafts reaction of a benzene derivative leading to ipso -substitution, a process that is energetically costly as it initially involves dearomatization of the benzene ring and generation of a highly congested quaternary carbon centre. Moreover, an intramolecular alkylation reaction could compete with retro-Michael addition (Firedel–Crafts). Notably, owing to the relatively weak C–Br (bond energy: 66 kcal mol −1 ) versus C–C bond (BDE of 83 versus 85 kcal mol −1 ), C–Br bond cleavage in alkylation process is more favourable than the retro-Michael reaction [54] . To verify this conclusion, studies were carried out with different arene-leaving groups using the same reaction conditions ( Table 4 ). As the results indicate, when the C–X bond energies (for example, C–H and C–O, Table 4 , entries 1 and 2) are larger than that of the C–C bond, retro-Michael addition is dominant and it results in no product formation. When C–X bond energies (for example, C–Br and C–I, entries 4 and 5) are smaller than that of the C–C bond, intramolecular cyclopropanation occurs and leads to a subsequent cascade that delivers product 3a . Table 4 The effects of leaving groups (X) on the fate of the arylation reactions. Full size table It is expected that reaction with chloro-arenes will not take place ( Table 4 , entry 3) as the C–Cl bond energy is close to that of the C–C bond, and the stronger electron-withdrawing ability of Cl would deactivate the aromatic system for the Friedel–Crafts reaction. In this effort, we have also prepared the stable p -acetoxy quinol 12 (see Supplementary Fig. S3 ). Treatment of 12 with trans -cinnamaldehyde ( 2a ) in the presence of catalyst I gives 4-acetyloxy phenol 13 and unreacted 2a . This finding indicates that retro-Michel (Friedel–Crafts) reaction via breaking of the weaker C–C bond rather than the stronger C–O bond prevails in this process. Taken together, the results described above not only provide support for the proposed reaction mechanism involving a Friedel–Crafts-initiated alkylation-ring opening cascade process but also can be used to explain why brominated arenes are critical for the success of the organocatalytic α-arylation reactions of enals. The mechanistic pathway outlined in Figure 3 also explains why at least 2 equiv of Na 2 CO 3 are important for the process. The base is required for the activation of the phenol for the initial Friedel–Crafts reaction (step 2). Furthermore, in step 4, it facilitates formation of enamine 9 for subsequent ring opening. The enamine-retro-Michael sequence has been demonstrated in our early studies of organocatalysed cyclopropanation reaction [38] . As observed earlier, treatment of the cyclopropane products with catalyst I in the presence of base (NaOAc) leads to ring opening to give enal products. The cross-coupling-like reaction is proposed to follow a similar pathway. The Michael adduct 7 proceeds an intramolecular alkylation through a favourable enol-exo-3-exo-tert attack to produce the strained spirocyclopropane intermediate 8 , which spontaneously undergoes formation of enamine 9 , followed by stereoselective retro-Michael reaction (ring opening) to give final product 3 with E configuration. Unlike the earlier cyclopropanation reaction, in the current process, isolation of the highly active intermediate cyclopropane aldehyde, derived from 8 , and species 7 and 9 is not possible. Interestingly, in situ 1 H NMR studies lead to the detection of resonance associated with the quinols 7 – 9 (see the procedure in Supporting Information and Supplementary Fig. S4 ) at 6.24–6.40, 6.50–6.58 and 6.61–6.68 p.p.m. Finally, the formation of major products 3 with ( E ) stereo configuration is consistent with the geometry of starting material trans -α,β-unsaturated aldehydes due to the essential orbital alignment for selective ring opening. In conclusion, in the effort described above, we have developed an unprecedented organocatalytic method for direct, stereoselective α-arylation of simple unfunctionalized α,β-unsaturated aldehydes. A novel iminium-initiated Michael-alkylation-enamine-ring-opening cascade process has been demonstrated by using mechanistic studies. The amine catalysed α-arylation reactions, which occur under mild conditions, display a broad substrate scope for the 4-bromophenols, 1-bromo-2-naphthol, 3-bromoindoles and α,β-unsaturated aldehyde reactants. Notably, synthetically challenging E -cross-coupling products are generated in good to high yields and with good to excellent levels of stereoselectivity. The conceptually novel cross-coupling strategy can also be viewed as a stereoselective C–H functionalization process using an organocatalyst [55] and, as such, adds a new process to the emerging field of organocatalysis. Finally, the unique transformation holds significant potential for applications to a broad spectrum of novel organic reactions, a proposal that will guide our further efforts in this area. General. 1 H (300 MHz) and 13 C (75 MHz) NMR spectra were recorded on a Bruker Avance 500. All commercially available reagents were used without further purification. The progress of the reactions was monitored by analytical thin-layer chromatography (TLC) on Whatman silica gel plates with fluorescence F 254 indicator. And Merck 60 silica gel was used for chromatography. Procedure for ( E )-α,β-diarylacrylaldehydes To a mixture of a substituted p -bromophenol ( 1a , 35 mg, 0.2 mmol), catalyst I (7 mg, 0.02 mmol) and Na 2 CO 3 (42 mg, 0.4 mmol) in 0.5 ml of chloroform at 60 °C was added a solution of a α,β-unsaturated aldehyde ( 2 , 0.1 mmol) in chloroform (1 ml) slowly via a syringe pump over 7 h. After the aldehyde was totally consumed (determined by TLC analysis), the vial was cooled to room temperature. The solvent was evaporated and the residue was purified by column chromatography, eluting with a mixture of ethyl acetate and hexane. The compound is characterized by 1 H and 13 C NMR and high-resolution mass spectrometry (HRMS) with >95% purity-based 1 H NMR. ( E )-2-(4-hydroxyphenyl)-3-(4-nitrophenyl)acrylaldehyde (3a) The title compound was prepared according to the typical procedure, as described above in 85% yield. Melting point (MP) 186–187 °C; 1 H NMR (acetone- d 6 , 500 MHz): δ =9.83 (s, 1H), 8.67 (br, 1H), 8.14 (d, J =8.5 Hz, 2H), 7.65 (s, 1H), 7.55 (d, J =8.5 Hz, 2H), 7.03 (d, J =8.5 Hz, 2H), 6.87 (d, J =8.5 Hz, 2H); 13 C NMR (acetone- d 6 , 125 MHz): δ =194.2, 158.6, 148.4, 146.3, 145.1, 142.1, 131.8, 131.6, 124.0, 116.3; HRMS (ESI) calcd. for C 15 H 11 NO 4 : m/z 292.0586 ([M+Na] + ), found 292.0583. ( E )-3-(4-fluorophenyl)-2-(4-hydroxyphenyl)acrylaldehyde (3b) The title compound was prepared according to the typical procedure as described above in 92% yield. 1 H NMR (acetone- d 6 , 500 MHz): δ =9.73 (s, 1H), 8.62 (br, 1H), 7.51 (s, 1H), 7.37 (m, 2H), 7.06 (t, J =9.0 Hz, 2H), 7.00 (d, J =8.5 Hz, 2H), 6.88 (d, J =8.5 Hz, 2H); 13 C NMR (acetone- d 6 , 125 MHz): δ =194.2, 164.8, 162.8, 158.1, 148.4, 142.4, 133.4, 133.3, 131.9, 131.4, 124.9, 116.2, 116.1, 115.9; HRMS (ESI) calcd. for C 15 H 11 FO 2 : m/z 265.0641 ([M+Na] + ), found 265.0640. ( E )-3-(4-chlorophenyl)-2-(4-hydroxyphenyl)acrylaldehyde (3c) The title compound was prepared according to the typical procedure as described above in 95% yield. 1 H NMR (acetone- d 6 , 500 MHz): δ =9.75 (s, 1H), 8.64 (br, 1H), 7.50 (s, 1H), 7.32 (s, 4H), 7.00 (d, J =8.5 Hz, 2H), 6.87 (d, J =9.0 Hz, 2H); 13 C NMR (acetone- d 6 , 125 MHz): δ =194.2, 158.2, 148.0, 143.1, 135.6, 134.3, 132.6, 131.4, 129.2, 124.7, 116.2; HRMS (ESI) calcd. for C 15 H 11 ClO 2 : m/z 281.0345 ([M+Na] + ), found 281.0339. ( E )-3-(4-bromophenyl)-2-(4-hydroxyphenyl)acrylaldehyde (3d) The title compound was prepared according to the typical procedure, as described above in 96% yield. MP 185–186 °C; 1 H NMR (acetone- d 6 , 500 MHz): δ =9.75 (s, 1H), 8.65 (br, 1H), 7.47 (m, 3H), 7.24 (d, J =8.5 Hz, 2H), 7.00 (d, J =8.5 Hz, 2H), 6.87 (d, J =8.5 Hz, 2H); 13 C NMR (acetone- d 6 , 125 MHz): δ =194.2, 158.3, 148.1, 143.2, 134.7, 132.8, 131.4, 124.7, 124.1, 116.3; HRMS (ESI) calcd. for C 15 H 11 BrO 2 : m/z 324.9840 ([M+Na] + ), found 324.9833. ( E )-4-(2-(4-hydroxyphenyl)-3-oxoprop-1-enyl)benzonitrile (3e) The title compound was prepared according to the typical procedure as described above in 86% yield. MP 160–162 °C; 1 H NMR (acetone- d 6 , 500 MHz): δ =9.80 (s, 1H), 8.64 (br, 1H), 7.69 (d, J =8.5 Hz, 2H), 7.58 (s, 1H), 7.48 (d, J =8.0 Hz, 2H), 7.01 (d, J =8.5 Hz, 2H), 6.87 (d, J =8.5 Hz, 2H); 13 C NMR (acetone- d 6 , 125 MHz): δ =194.2, 158.5, 146.9, 144.7, 140.1, 132.8, 131.5, 128.7, 124.2, 118.8, 116.3, 115.8, 113.1; HRMS (ESI) calcd. for C 16 H 11 NO 2 : m/z 272.0687 ([M+Na] + ), found 272.0681. ( E )-3-(3-fluorophenyl)-2-(4-hydroxyphenyl)acrylaldehyde (3f) The title compound was prepared according to the typical procedure as described above in 62% yield. 1 H NMR (acetone- d 6 , 500 MHz): δ =9.77 (s, 1H), 8.60 (br, 1H), 7.53 (s, 1H), 7.34 (m, 1H), 7.18 (d, J =8.0 Hz, 1H), 7.10 (m, 1H), 7.01 (m, 3H), 6.89 (d, J =8.5 Hz, 2H); 13 C NMR (acetone- d 6 , 125 MHz): δ =194.3, 158.4, 147.9, 143.7, 137.9, 131.4, 131.1, 131.0, 127.4, 124.7, 117.2, 117.1, 117.0, 116.3; HRMS (ESI) calcd. for C 15 H 11 FO 2 : m/z 265.0641 ([M+Na] + ), found 265.0636. ( E )-3-(2-fluorophenyl)-2-(4-hydroxyphenyl)acrylaldehyde (3g) The title compound was prepared according to the typical procedure as described above in 77% yield. MP 165–166 °C; 1 H NMR (acetone- d 6 , 500 MHz): δ =9.83 (s, 1H), 8.56 (br, 1H), 7.62 (s, 1H), 7.37 (m, 1H), 7.19 (m, 1H), 7.02 (m, 4H), 6.85 (d, J =8.5 Hz, 2H); 13 C NMR (acetone- d 6 , 125 MHz): δ =194.2, 158.3, 144.0, 140.5, 140.4, 132.5, 132.4, 131.5, 131.0, 124.6, 116.5, 116.3, 116.1; HRMS (ESI) calcd. for C 15 H 11 FO 2 : m/z 265.0641 ([M+Na] + ), found 265.0642. ( E )-3-(2-chlorophenyl)-2-(4-hydroxyphenyl)acrylaldehyde (3h) The title compound was prepared according to the typical procedure as described above in 69% yield. 1 H NMR (acetone- d 6 , 500 MHz): δ =9.87 (s, 1H), 8.58 (br, 1H), 7.68 (s, 1H), 7.50 (d, J =8.0 Hz, 1H), 7.31 (m, 1H), 7.06 (m, 2H), 6.98 (d, J =9.0 Hz, 2H), 6.80 (d, J =8.5 Hz, 2H); 13 C NMR (acetone- d 6 , 125 MHz): δ =194.2, 158.2, 145.0, 144.0, 134.9, 134.1, 131.7, 131.6, 131.3, 130.3, 127.2, 124.0, 115.9; HRMS (ESI) calcd. for C 15 H 11 ClO 2 : m/z 281.0345 ([M+Na] + ), found 281.0337. ( E )-2-(4-hydroxyphenyl)-3-phenylacrylaldehyde (3i) The title compound was prepared according to the typical procedure as described above in 99% yield. MP 152–153 °C; 1 H NMR (acetone- d 6 , 500 MHz): δ =9.72 (s, 1H), 8.55 (br, 1H), 7.47 (s, 1H), 7.25 (m, 5H), 6.97 (d, J =8.5 Hz, 2H), 6.84 (d, J =8.5 Hz, 2H); 13 C NMR (acetone- d 6 , 125 MHz): δ =194.3, 158.0, 149.8, 142.6, 135.4, 131.4, 131.1, 130.4, 129.0, 125.1, 116.1; HRMS (ESI) calcd. for C 15 H 12 O 2 : m/z 247.0735 ([M+Na] + ), found 247.0733. ( E )-2-(4-hydroxyphenyl)-3-(4-methoxyphenyl)acrylaldehyde (3j) The title compound was prepared according to the typical procedure, as described above in 99% yield. MP 180–181 °C; 1 H NMR (acetone- d 6 , 500 MHz): δ =9.68 (s, 1H), 8.57 (br, 1H), 7.43 (s, 1H), 7.27 (d, J =9.0 Hz, 2H), 7.00 (d, J =8.5 Hz, 2H), 6.88 (d, J =8.5 Hz, 2H), 6.83 (d, J =9.0 Hz, 2H); 13 C NMR (acetone- d 6 , 125 MHz): δ =194.1, 161.9, 157.9, 149.9, 140.7, 133.1, 131.4, 127.9, 125.6, 116.2, 114.5, 55.5; HRMS (ESI) calcd. for C 16 H 14 O 3 : m/z 277.0841 ([M+Na] + ), found 277.0838. ( E )-2-(4-hydroxyphenyl)-3- p -tolylacrylaldehyde (3k) The title compound was prepared according to the typical procedure as described above in 99% yield. MP 188–190 °C; 1 H NMR (acetone- d 6 , 500 MHz): δ =9.72 (s 1H), 8.56 (br, 1H), 7.46 (s, 1H), 7.20 (d, J =8.5 Hz, 2H), 7.09 (d, J =8.0 Hz, 2H), 7.00 (d, J =8.5 Hz, 2H), 6.87 (d, J =8.5 Hz, 2H), 2.28 (s, 3H); 13 C NMR (acetone- d 6 , 125 MHz): δ =194.3, 158.0, 150.0, 141.9, 140.9, 132.6, 131.4, 131.2, 129.7, 125.4, 116.1, 21.1; HRMS (ESI) calcd. for C 16 H 14 O 2 : m/z 261.0891 ([M+Na] + ), found 261.0888. Procedure for ( E) -α-indolyl-β-arylacrylaldehyde 3-Bromoindole ( 4 , 39 mg, 0.2 mmol), α,β-unsaturated aldehyde ( 2 , 0.1 mmol), NaOAc (42 mg, 0.4 mmol) and catalyst I (20 mmol%, 7 mg, 0.02 mmol) were dissolved in chloroform (0.2 M relative to aldehyde, 0.5 ml) at room temperature, and the reaction mixture were heated to 60 °C. After the aldehyde was totally consumed (determined by TLC analysis), the vial was cooled to room temperature. The solvent was evaporated and the residue was purified by column chromatography, eluting with a mixture of ethyl acetate and hexane. The compound is characterized by 1 H and 13 C NMR and HRMS with >95% purity-based 1 H NMR. ( E )-2-(1 H -indol-3-yl)-3-(4-nitrophenyl)acrylaldehyde (5a) The title compound was prepared according to the typical procedure as described above in 90% yield. MP 211–212 °C; 1 H NMR (acetone- d 6 , 500 MHz): δ =10.82 (br, 1H), 9.93 (s, 1H), 8.04 (d, J =9.0 Hz, 2H), 7.69 (s, 1H), 7.62 (m, 3H), 7.48 (d, J =8.0 Hz, 1H), 7.07 (t, J =7.5, 1H), 6.81 (t, J =7.5, 1H), 6.74 (d, J =8.0 Hz, 1H); 13 C NMR (acetone- d 6 , 125 MHz): δ =194.7, 148.3, 144.4, 143.2, 138.3, 137.6, 131.7×2, 128.3, 125.7, 124.1×2, 122.7, 121.0, 120.4, 112.8, 107.1; HRMS (ESI) calcd. for C 17 H 12 N 2 O 3 : m/z 315.0746 ([M+Na] + ), found 315.0742. ( E )-3-(4-chlorophenyl)-2-(1 H -indol-3-yl)acrylaldehyde (5b) The title compound was prepared according to the typical procedure as described above in 79% yield. 1 H NMR (acetone- d 6 , 500 MHz): δ =10.65 (br, 1H), 9.86 (s, 1H), 7.60 (s, 1H), 7.53 (s, 1H), 7.47 (d, J =8 Hz, 1H), 7.41 (d, J =8.5 Hz, 2H), 7.23 (d, J =8.5 Hz, 2H), 7.08 (t, J =7.5 Hz, 1H), 6.90–6.81 (m, 2H); 13 C NMR (acetone- d 6 , 125 MHz): δ =194.6, 146.8, 137.4, 136.1, 135.3, 135.2, 132.4×2, 129.1×2, 127.4, 125.8, 122.3, 120.9, 120.0, 112.5, 107.3; HRMS (ESI) calcd. for C 17 H 12 ClNO: m/z 304.0505 ([M+Na] + ), found 304.0503. ( E )-3-(4-bromophenyl)-2-(1 H -indol-3-yl)acrylaldehyde (5c) The title compound was prepared according to the typical procedure as described above in 100% yield. 1 H NMR (acetone- d 6 , 500 MHz): δ =10.65 (br, 1H), 9.86 (s, 1H), 7.58 (s, 1H), 7.53 (s, 1H), 7.47 (d, J =8 Hz, 1H), 7.39–7.33 (m, 4H), 7.08 (t, J =7.5 Hz, 1H), 6.87–6.82 (m, 2H); 13 C NMR (acetone- d 6 , 125 MHz): δ =194.6, 146.8, 137.4, 136.1, 135.5, 132.6×2, 132.1×2, 127.4, 125.8, 123.7, 122.3, 120.9, 120.0, 112.5, 107.3; HRMS (ESI) calcd. for C 17 H 12 BrNO: m/z 348.0000 ([M+Na] + ), found 347.9993. ( E )-4-(2-(1 H -indol-3-yl)-3-oxoprop-1-enyl)benzonitrile (5d) The title compound was prepared according to the typical procedure as described above in 81% yield. MP 232–234 °C; 1 H NMR (acetone- d 6 , 500 MHz): δ =10.74 (br, 1H), 9.91 (s, 1H), 7.65 (s, 1H), 7.60–7.55 (m, 5H), 7.47 (d, J =8 Hz, 1H), 7.08 (t, J =7.5 Hz, 1H), 6.83 (t, J =7.5 Hz, 1H), 6.75 (d, J =8 Hz, 1H); 13 C NMR (acetone- d 6 , 125 MHz): δ =194.7, 145.2, 141.1, 137.8, 137.5, 132.7×2, 131.4×2, 128.1, 125.7, 122.6, 120.9, 120.3, 119.1, 112.8, 112.7, 107.1; HRMS (ESI) calcd. for C 18 H 12 N 2 O: m/z 295.0847 ([M+Na] + ), found 295.0841. ( E )-3-(2-chlorophenyl)-2-(1 H -indol-3-yl)acrylaldehyde (5e) The title compound was prepared according to the typical procedure as described above in 100% yield. 1 H NMR (CDCl 3 , 500 MHz): δ =9.92 (s, 1H), 8.49 (br, 1H), 7.72 (s, 1H), 7.52–7.43 (m, 2H), 7.33 (d, J =8 Hz, 1H), 7.15–7.09 (m, 3H), 6.88 (t, J =7.5 Hz, 1H), 6.82–6.79 (m, 2H); 13 C NMR (CDCl 3 , 125 MHz): δ =194.9, 144.7, 136.3, 136.0, 134.9, 134.0, 130.8, 130.7, 129.9, 126.8, 126.7, 125.1, 122.5, 120.8, 120.3, 111.5, 107.2; HRMS (ESI) calcd. for C 17 H 12 ClNO: m/z 304.0505 ([M+Na] + ), found 304.0503. ( E )-3-(2-bromophenyl)-2-(1 H -indol-3-yl)acrylaldehyde (5f) The title compound was prepared according to the typical procedure, as described above in 100% yield. 1 H NMR (CDCl 3 , 500 MHz): δ =9.93 (s, 1H), 8.46 (br, 1H), 7.65 (d, J =8 Hz, 1H), 7.64 (s, 1H), 7.44 (s, 1H), 7.33 (d, J =8 Hz, 1H), 7.11–7.09 (m, 2H), 7.05 (t, J =7.5, 1H), 6.89–6.80 (m, 3H); 13 C NMR (CDCl 3 , 125 MHz): δ =194.8, 147.06, 136.3, 135.9, 133.1, 131.0, 130.7, 127.4, 127.2, 126.6, 125.4, 125.1, 122.5, 120.9, 120.3, 111.5, 107.2; HRMS (ESI) calcd. for C 17 H 12 BrNO: m/z 348.0000 ([M+Na] + ), found 347.9996. ( E )-2-(1 H -indol-3-yl)-3-phenylacrylaldehyde (5g) The title compound was prepared according to the typical procedure as described above in 87% yield. MP 126–127 °C; 1 H NMR (CDCl 3 , 500 MHz): δ =10.15 (s, 1H), 9.86 (br, 1H), 7.53 (s, 1H), 7.40–7.35 (m, 4H), 7.25 (m, 1H), 7.19–7.13 (m, 3H), 6.94–6.90 (m, 2H); 13 C NMR (CDCl 3 , 125 MHz): δ =195.1, 149.8, 136.4, 135.2, 134.6, 130.7×2, 130.1, 128.6×2, 125.9, 125.4, 122.5, 121.0, 120.2, 111.6, 107.8; HRMS (ESI) calcd. for C 17 H 13 NO: m/z 270.0895 ([M+Na] + ), found 270.0892. ( E )-2-(1 H -indol-3-yl)-3-(4-methoxyphenyl)acrylaldehyde (5h) The title compound was prepared according to the typical procedure, as described above in 75% yield. 1 H NMR (CDCl 3 , 500 MHz): δ =9.80 (s, 1H), 8.52 (br, 1H), 7.44 (s, 1H), 7.38 (d, J =8.0 Hz, 1H), 7.32 (s, 1H), 7.31 (d, J =8.5 Hz, 2H), 7.16 (t, J =7.5 Hz, 1H), 7.00 (d, J =8.0 Hz, 1H), 6.95 (t, J =7.5 Hz, 1H), 6.69 (d, J =8.5 Hz, 2H), 3.77 (s, 3H); 13 C NMR (CDCl 3 , 125 MHz): δ =195.1, 161.3, 150.2, 136.4, 132.8×2, 132.5, 127.9, 125.6×2, 122.4, 121.0, 121.2, 114.1×2, 111.6, 108.1, 55.5; HRMS (ESI) calcd. for C 18 H 15 NO 2 : m/z 300.1000 ([M+Na] + ), found 300.0995. ( E )-2-(1 H -indol-3-yl)-3-p-tolylacrylaldehyde (5i) The title compound was prepared according to the typical procedure, as described above in 90% yield. MP 159–160 °C; 1 H NMR (CDCl 3 , 500 MHz): δ =9.83 (s, 1H), 8.49 (br, 1H), 7.46 (s, 1H), 7.38 (d, J =8 Hz, 1H), 7.34 (d, J =2.5 Hz, 1H), 7.25 (d, J =8 Hz, 2H), 7.15 (t, J =7.5 Hz, 1H), 6.99–6.92 (m, 4H), 2.28 (s, 3H); 13 C NMR (CDCl 3 , 125 MHz): δ =195.1, 150.3, 140.7, 136.4, 133.7, 132.4, 130.9×2, 129.4×2, 125.7, 125.5, 122.4, 121.1, 120.2, 111.6, 108.0, 21.8; HRMS (ESI) calcd. for C 18 H 15 NO: m/z 284.1051 ([M+Na] + ), found 284.1047. ( E )-2-(1 H -indol-3-yl)-3-(2-methoxyphenyl)acrylaldehyde (5j) The title compound was prepared according to the typical procedure as described above in 89% yield. MP 167–168 °C; 1 H NMR (CDCl 3 , 500 MHz): δ =9.88 (s, 1H), 8.47 (br, 1H), 7.87 (s, 1H), 7.38 (d, J =2.5 Hz, 1H), 7.34 (d, J =8 Hz, 1H), 7.21 (t, J =7.8 Hz, 1H), 7.13–7.10 (m, 2H), 6.97–6.88 (m, 3H), 6.52 (t, J =7.8 Hz, 1H), 3.94 (s, 3H); 13 C NMR (CDCl 3 , 125 MHz): δ =195.4, 158.1, 144.5, 136.4, 134.2, 131.5, 130.3, 125.9, 125.3, 124.4, 122.3, 121.1, 120.4, 120.0, 111.5, 110.8, 108.1, 55.9; HRMS (ESI) calcd. for C 18 H 15 NO 2 : m/z 300.1000 ([M+Na] + ), found 300.0999. ( E )-2-(1 H -indol-3-yl)-3- o -tolylacrylaldehyde (5k) The title compound was prepared according to the typical procedure as described above in 97% yield. 1 H NMR (CDCl 3 , 500 MHz): δ =9.90 (s, 1H), 8.40 (br, 1H), 7.61 (s, 1H), 7.40 (d, J =2.5 Hz, 1H), 7.33 (d, J =8.5 Hz, 1H), 7.23 (d, J =7.5 Hz, 1H), 7.14–7.08 (m, 3H), 6.85 (t, J =7.5 Hz, 1H), 6.80–6.77 (m, 2H), 2.50 (s, 3H); 13 C NMR (CDCl 3 , 125 MHz): δ =195.0, 147.4, 137.6, 136.3, 135.3, 134.7, 130.6, 129.6, 129.4, 126.3, 125.9, 125.3, 122.3, 121.0, 120.1, 111.4, 107.9, 20.5; HRMS (ESI) calcd. for C 18 H 15 NO: m/z 284.1051 ([M+Na] + ), found 284.1046. ( E )-4-(2-(1 H -indol-3-yl)-3-oxoprop-1-enyl)-2-methoxyphenyl acetate (5l) The title compound was prepared according to the typical procedure as described above in 94% yield. 1 H NMR (CDCl 3 , 500 MHz): δ =9.85 (s, 1H), 8.57 (br, 1H), 7.44 (s, 1H), 7.36 (d, J =8, 1H), 7.30 (s, 1H), 7.14 (t, J =7.5 Hz, 1H), 7.06 (d, J =8 Hz, 1H), 7.00–6.95 (m, 3H), 6.85 (s, 1H), 3.02 (s, 3H), 2.26 (s, 3H); 13 C NMR (CDCl 3 , 125 MHz): δ =195.0, 169.0, 150.8, 148.9, 141.2, 136.3, 134.4, 133.8, 125.8, 125.3, 124.8, 122.8, 122.7, 121.1, 120.4, 114.1, 111.6, 107.6, 55.2, 20.9; HRMS (ESI) calcd. for C 20 H 17 NO 4 : m/z 358.1055 ([M+Na] + ), found 358.1053. ( E )-3-(furan-2-yl)-2-(1 H -indol-3-yl)acrylaldehyde (5m) The title compound was prepared according to the typical procedure as described above in 90% yield. 1 H NMR (CDCl 3 , 500 MHz): δ =9.78 (s, 1H), 8.49 (br, 1H), 7.47 (s, 1H), 7.43 (d, J =8 Hz, 1H), 7.40 (s, 1H), 7.36 (d, J =2.5 Hz, 1H), 7.20 (t, J =7.5 Hz, 1H), 7.15 (d, J =8 Hz, 1H), 7.04 (t, J =7.5 Hz, 1H), 6.32–6.31 (m, 1H), 6.20 (d, J =3.5 Hz, 1H); 13 C NMR (CDCl 3 , 125 MHz): δ =193.8, 151.4, 145.4, 136.3, 136.0, 131.3, 125.6, 125.5, 122.5, 121.0, 120.2, 116.8, 113.1, 111.7, 107.9; HRMS (ESI) calcd. for C 15 H 11 NO 2 : m/z 260.0687 ([M+Na] + ), found 260.0684. ( E )-2-(1 H -indol-3-yl)-3-(naphthalen-2-yl)acrylaldehyde (5n) The title compound was prepared according to the typical procedure as described above in 78% yield. 1 H NMR (CDCl 3 , 500 MHz): δ =9.91 (s, 1H), 8.49 (br, 1H), 7.94 (s, 1H), 7.71–7.69 (m, 2H), 7.65 (s, 1H), 7.51–7.40 (m, 5H), 7.35 (d, J =9 Hz, 1H), 7.14 (t, J =7.5 Hz, 1H), 6.97 (d, J =8 Hz, 1H), 6.87 (t, J =7.5 Hz, 1H); 13 C NMR (CDCl 3 , 125 MHz): δ =195.0, 149.7, 136.4, 134.6, 134.0, 133.3, 133.0, 132.0, 128.9, 128.0, 127.9, 127.6, 126.8, 126.7, 126.0, 125.7, 122.6, 121.1, 120.3, 111.6, 108.; HRMS (ESI) calcd. for C 21 H 15 NO: m/z 320.1051 ([M+Na] + ), found 320.1050. 10 H -furo[3,2-a]carbazole-5-carbaldehyde (S5) A solution of Boc-protected 5m (67 mg, 0.2 mmol) dissolved in acetone (7 ml) in the presence of a catalytic amount of I 2 was irradiated for 12 h in a reactor with an HPK-125W Philips high-pressure mercury vapour UV lamp in a water-jacketed immersion well. The solvent was evaporated and the residue was purified by chromatography on silica gel in 55% yield. MP decomposed >258 °C; 1 H NMR (acetone- d 6 , 500 MHz): δ =11.29 (br, 1H), 10.50 (s, 1H), 9.13 (d, J =8.5 Hz, 1H), 8.17 (s, 1H), 8.09 (s, 1H), 7.62 (d, J =8.0 Hz, 1H), 7.45 (t, J =7.5 Hz, 1H), 7.38 (s, 1H), 7.26 (t, J =7.5 Hz, 1H); 13 C NMR (acetone- d 6 , 125 MHz): δ =193.1, 154.2, 149.2, 141.1, 134.6, 130.0, 126.4, 126.1, 123.8, 120.3, 118.6, 116.1, 112.6, 111.8, 105.6; HRMS (ESI) calcd. for C 15 H 9 NO 2 : m/z 258.0531 ([M+Na] + ), found 258.0528. 1 H NMR study of the formation of quinols Trans - p -nitro-cinnamaldehyde ( 2a , 18 mg, 0.1 mmol) and 4-bromophenol ( 1a , 26 mg, 0.15 mmol) and catalyst I (0.02 mmol) were dissolved in 0.8 ml of CDCl 3 and the reaction mixture was transferred into a NMR tube. A small magnetic stir bar was used to stir the mixture, and it was removed before 1 H NMR measurement. The reaction mixture was monitored with designated period of time (2, 8, 10, 49 h, and 3 days). How to cite this article: Song, X. et al . Direct stereoselective α-arylation of unmodified enals using an organocatalytic cross-coupling-like reaction. Nat. Commun. 2:524 doi: 10.1038/ncomms1541 (2011).